Src activation by β-adrenoreceptors is a key switch for tumour metastasis Noradrenaline can modulate multiple cellular functions important for cancer progression; however, how this single extracellular signal regulates such a broad array of cellular processes is unknown. Here we identify Src as a key regulator of phosphoproteomic signalling networks activated in response to beta-adrenergic signalling in cancer cells. These results also identify a new mechanism of Src phosphorylation that mediates beta-adrenergic/PKA regulation of downstream networks, thereby enhancing tumour cell migration, invasion and growth. In human ovarian cancer samples, high tumoural noradrenaline levels were correlated with high pSrc Y419 levels. Moreover, among cancer patients, the use of beta blockers was significantly associated with reduced cancer-related mortality. Collectively, these data provide a pivotal molecular target for disrupting neural signalling in the tumour microenvironment. The tumour microenvironment is an important determinant of cancer progression, and microenvironmental distribution of neural and endocrine signals has now been identified as a key mediator of these dynamics [1] , [2] . For example, signalling resulting from activation of beta-adrenergic receptors (ADRB) by noradrenaline (NA) affects a broad array of processes involved in the progression of various cancer types [1] , [2] . However, the diversity of intracellular signalling pathways and cellular processes modulated by this single extracellular signal is surprising. For example, our previous work determined that sympathetic nervous system activity can directly enhance the pathogenesis of ovarian carcinoma by protecting tumour cells from anoikis [3] , promoting tumour cell invasion [4] , [5] , [6] and tumour-associated angiogenesis [2] , [7] . We found that these effects were mediated through activation of tumour cell ADRB2, but its downstream signalling pathways are not well understood. Here, we sought to determine key regulators of the cellular phosphoproteome following NA stimulation of ADRB in cancer cells. We demonstrate that ADRB signalling leads to Src activation by a unique PKA-mediated mechanism, which is critical to the regulation of phosphoproteomic networks associated with ovarian cancer progression. NA activated signalling networks Following treatment of SKOV3ip1 cells with NA, proteins from treated and untreated cells were separated by 2D gel electrophoresis and stained for total and phosphorylated proteins ( Supplementary Fig. S1a,b ). Quantitative analyses of these samples, followed by mass spectrometry analysis identified 24 proteins with altered expression levels and 39 with differential phosphorylation ( Supplementary Tables S1 and 2 and Supplementary Data 1 and 2 ). For each of these proteins, we identified kinases that may be upstream by up to two levels (the kinase targets another kinase, which targets the protein). To identify putative key mediators, all involved kinases were scored by the number of identified downstream proteins. The highest score was achieved for Src ( Fig. 1 and Supplementary Fig. S2a ). To validate this finding, lysates from NA-treated tumour cells were subjected to immunoblotting, which confirmed the results obtained in our analysis ( Supplementary Fig. S2b ). Additionally, treatment with either dasatinib or Src small interfering RNA (siRNA) abrogated NA-induced changes ( Supplementary Fig. S2b ). Next, we sought to determine the functional and biological roles of Src in promoting tumour growth in response to increased adrenergic signalling. 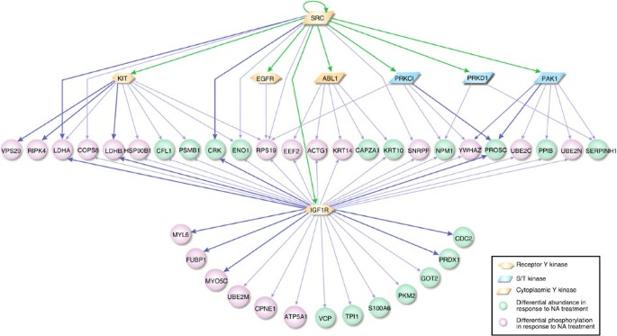Figure 1: Putative phosphorylation cascade triggered by the NA-induced activation of Src. In this predicted network (see ‘Signaling Network Analysis’ in ‘Methods’), the components connecting Src to the NA-responsive proteins are shown as arrows: green, experimentally observed phosphorylation according to PhosphoELM; dark blue, predicted by NetworKIN; light blue, predicted by NetworKIN for a close homologue of the target. Figure 1: Putative phosphorylation cascade triggered by the NA-induced activation of Src. In this predicted network (see ‘Signaling Network Analysis’ in ‘ Methods ’), the components connecting Src to the NA-responsive proteins are shown as arrows: green, experimentally observed phosphorylation according to PhosphoELM; dark blue, predicted by NetworKIN; light blue, predicted by NetworKIN for a close homologue of the target. Full size image Beta-adrenergic receptors mediate NA-induced Src activation We first examined Y419 phosphorylation following NA stimulation. As ovarian cancer cells do not produce NA (data not shown), we exposed cells to various NA concentrations known to be present in ovarian tissues and tumours under physiological and stress conditions [2] , [8] . In the ADRB-positive HeyA8 and SKOV3ip1 human ovarian cancer cells [2] , [9] , pSrc Y419 levels increased markedly (at least three-fold) following exposure to 100 nM–10 μM NA ( Fig. 2a and Supplementary Fig. S3a ). These increases are comparable to those seen by growth factor-mediated Src phosphorylation, as observed in Supplementary Fig. S3b . To show that Y419 phosphorylation leads to Src activation, we performed a kinase assay where focal adhesion kinase (FAK) was exposed to Src or a combination of Src with AP23846. Upon interaction with Src, FAK Y397 phosphorylation was substantially increased, while AP23846 blocked this effect ( Supplementary Fig. S3c ). Additionally, we show that FAK exposure to Src results in increased phosphorylation at Y925 that is not seen in the absence of ATP ( Supplementary Fig. S3c ). Similar responses to NA with regard to Y419 phosphorylation were noted with ADRB-positive breast cancer and melanoma cell lines ( Supplementary Fig. S3d ). In contrast, NA stimulation of the ADRB-deficient A2780-PAR cells [2] or hydrocortisone treatment of SKOV3ip1 cells did not increase pSrc Y419 levels ( Supplementary Fig. S3e and data not shown). Propranolol blocked NA-mediated Src activation ( Supplementary Fig. S3e ). Given the known role of pSrc Y530 dephosphorylation in Src activation, we also probed for pSrc Y530 following NA stimulation. There was no change in pSrc Y530 phosphorylation, suggesting that the NA-induced Src activation was solely mediated by phosphorylation at Y419 ( Supplementary Fig. S3f,g ). To further corroborate these findings, HeyA8 cells were treated with isoproterenol (10 μM), which resulted in Src Y419 phosphorylation within 5 min ( Supplementary Fig. S3h ). Butoxamine, blocked the NA-induced Src activation ( Fig. 2b ). To examine the specificity of ADRB receptors in mediating NA-induced activation of Src, we utilized ADRB1- or ADRB2-targeted siRNA capable of reducing levels of each protein by >80% ( Supplementary Fig. S3i ). Similar to the effects with inhibitors, ADRB1 and ADRB2 siRNA abrogated NA-induced Src activation ( Fig. 2c ). Next, we created stable clones of A2780-PAR cells transfected with an ADRB2 construct. After confirming ADRB2 expression ( Supplementary Fig. S3j ), we treated these cells with NA, which resulted in increased Src Y419 phosphorylation ( Supplementary Fig. S3k ). 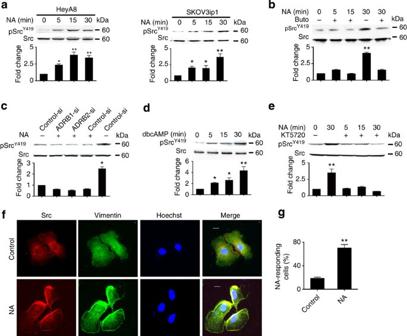Figure 2: NA-induced Src activation is mediated by an ADRB/cAMP/PKA mechanism. (a) Effect of 10 μM NA on SrcY419phosphorylation in HeyA8 and SKOV3ip1 cells. *P<0.01, **P<0.001; two-tail Student’st-test. (b) HeyA8 cells were incubated for 1 h with 1 μM butoxamine (Buto, β2antagonist), exposed to 10 μM NA and probed for pSrcY419. *P<0.001; two-tail Student’st-test. (c) Similar experiments were performed with siRNA targeted against ADRB1 (ADRB1 si) or ADRB2 (ADRB2 si) in SKOV3ip1 cells. *P<0.001; two-tail Student’st-test. (d) Effect of 50 μM dbcAMP (PKA agonist) on pSrcY419in SKOV3ip1 cells. *P<0.01, **P<0.001; two-tail Student’st-test. (e) HeyA8 cells were exposed to 10 μM KT5720 (PKA antagonist) for 1 h, stimulated with 10 μM NA and probed for pSrcY419. *P<0.001; two-tail Student’st-test. (f) SKOV3ip1 cells were treated with 10 μM NA, and Src was visualized by immunofluorescence (scale bar, 9.375 μm). (g) Quantification of cellular response to NA (measured as cells with increased Src expression at the focal adhesions) is shown in graphs *P<001; two-tail Student’st-test. In panels (a–e), the immunoblot is shown at the top and quantification of pSrc band intensity relative to the intensity of the total Src band is shown below. Figure 2: NA-induced Src activation is mediated by an ADRB/cAMP/PKA mechanism. ( a ) Effect of 10 μM NA on Src Y419 phosphorylation in HeyA8 and SKOV3ip1 cells. * P <0.01, ** P <0.001; two-tail Student’s t -test. ( b ) HeyA8 cells were incubated for 1 h with 1 μM butoxamine (Buto, β 2 antagonist), exposed to 10 μM NA and probed for pSrc Y419 . * P <0.001; two-tail Student’s t -test. ( c ) Similar experiments were performed with siRNA targeted against ADRB1 (ADRB1 si) or ADRB2 (ADRB2 si) in SKOV3ip1 cells. * P <0.001; two-tail Student’s t -test. ( d ) Effect of 50 μM dbcAMP (PKA agonist) on pSrc Y419 in SKOV3ip1 cells. * P <0.01, ** P <0.001; two-tail Student’s t -test. ( e ) HeyA8 cells were exposed to 10 μM KT5720 (PKA antagonist) for 1 h, stimulated with 10 μM NA and probed for pSrc Y419 . * P <0.001; two-tail Student’s t -test. ( f ) SKOV3ip1 cells were treated with 10 μM NA, and Src was visualized by immunofluorescence (scale bar, 9.375 μm). ( g ) Quantification of cellular response to NA (measured as cells with increased Src expression at the focal adhesions) is shown in graphs * P <001; two-tail Student’s t -test. In panels ( a – e ), the immunoblot is shown at the top and quantification of pSrc band intensity relative to the intensity of the total Src band is shown below. Full size image NA-induced Src activation is mediated by cAMP/PKA We next performed a series of experiments to delineate the signalling pathway involved in NA-mediated Src activation. Treatment of SKOV3ip1 cells with forskolin resulted in rapid Src Y419 phosphorylation ( Supplementary Fig. S3l ). To test whether PKA was involved in NA-mediated Src activation, cells were treated with dibutyryl-cAMP (dbcAMP), resulting in rapid Src Y419 phosphorylation ( Fig. 2d ). Furthermore, PKA silencing by siRNA or PKA inhibitors prevented NA-mediated Src activation ( Fig. 2e and Supplementary Fig. S3m,n ). Immunofluorescence analyses verified that upon NA stimulation, Src localizes to the focal adhesions in SKOV3ip1 cells ( Fig. 2f and Supplementary Fig. S3o ). pSrc S17 is required for NA-induced Src activation As PKA is a serine-threonine kinase, the paradoxical increase in Src tyrosine phosphorylation prompted us to consider potential underlying mechanisms. Src contains a single consensus PKA site at residues surrounding S17 ( Supplementary Fig. S4a ) [10] . To test whether NA and dbcAMP-mediated induction of Src S17 phosphorylation was PKA-dependent, we treated HeyA8 cells with NA or dbcAMP. Both treatments rapidly increased pSrc S17 levels ( Fig. 3a and Supplementary Fig. S4b ). Furthermore, in ADRB2-null A2780-PAR cells stably transfected with ADRB2, NA stimulation rapidly increased PKA activity, Src S17 phosphorylation and Src activation ( Supplementary Fig. S4c,d ). To determine whether Ser17 phosphorylation is a prerequisite for NA-induced Src Y419 phosphorylation, mouse embryonic fibroblast cells null for Src, Yes or Fyn (SYF) were transfected with plasmids containing either wild-type (WT) Src or Src mutated at S17 (S17A). To verify that NA could increase PKA activity in SYF cells, we measured phospho-PKA substrate levels in these cells. As expected, NA rapidly increased the levels of phospho-PKA substrates ( Supplementary Fig. S3e ). In addition, after verifying the transfection efficiency and confirming that WT and S17A Src were transiently expressed at similar levels ( Supplementary Fig. S4f,g ), we exposed them to NA or dbcAMP. Src Y419 and Src S17 were rapidly phosphorylated in WT Src-expressing cells following NA treatment, but not in the S17A Src-transfected cells ( Fig. 3b and Supplementary Fig. S4h ). 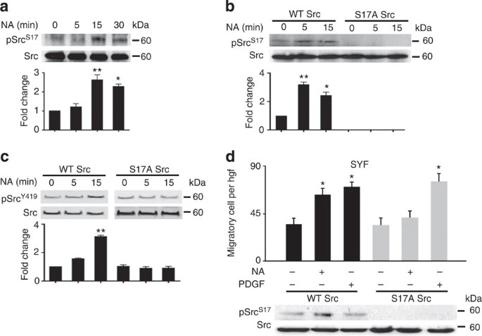Figure 3: NA-induced SrcS17phosphorylation on SYF cells is required for Src activation. (a) HeyA8 cells were treated with 10 μM NA and probed for pSrcS17. *P<0.01; **P<0.001; two-tail Student’st-test. SYF-null cells transfected with either WT or mutant Src (S17A) were stimulated with 10 μM NA and immunoblotted for (b) pSrcS17or (c) pSrcY419. *P<0.01; **P<0.001; two-tail Student’st-test. (d) SYF-null cells transfected with either WT or mutant Src (S17A) were stimulated with 10 μM NA or PDGF (20 ng ml−1) and subjected to a migration assay or western blot analysis for pSrcS17expression. *P<0.01; two-tail Student’st-test. In panels (a–c), the immunoblot is shown at the top and quantification of pSrc band intensity relative to the intensity of the total Src band is shown below. Figure 3: NA-induced Src S17 phosphorylation on SYF cells is required for Src activation. ( a ) HeyA8 cells were treated with 10 μM NA and probed for pSrc S17 . * P <0.01; ** P <0.001; two-tail Student’s t -test. SYF-null cells transfected with either WT or mutant Src (S17A) were stimulated with 10 μM NA and immunoblotted for ( b ) pSrc S17 or ( c ) pSrc Y419 . * P <0.01; ** P <0.001; two-tail Student’s t -test. ( d ) SYF-null cells transfected with either WT or mutant Src (S17A) were stimulated with 10 μM NA or PDGF (20 ng ml −1 ) and subjected to a migration assay or western blot analysis for pSrc S17 expression. * P <0.01; two-tail Student’s t -test. In panels ( a – c ), the immunoblot is shown at the top and quantification of pSrc band intensity relative to the intensity of the total Src band is shown below. Full size image Interaction between pS17 and Src exposes Y419 The contribution of the Src N-terminus, where S17 resides, and specifically its unique domain to Src activation is not known, as the reported Src crystal structure does not include the first 82 amino-acid residues [11] . To understand how S17 phosphorylation might lead to subsequent Y419 phosphorylation, we performed molecular dynamic simulations. First, we obtained the atomic coordinates of c-Src from the Protein Data Bank (Code: 2SRC ) [12] , and proceeded to eliminate phospho-aminophosphonic acid-adenylate ester (ANP) and water molecules, leaving Src in its inactive form ( Fig. 4a ). Subsequently, we ran preliminary simulations with a computer designed full-length N-terminal attached to the known Src crystal structure. After performing extensive annealing molecular dynamic simulations, no significant data in the time scale of the simulation could be obtained (data not shown). Next, we constructed a model peptide that resembled the N-terminus where Ser17 resides (K9-E19 fragment). An initial estimate of the secondary structure was generated using the PSIPRED server and submitted to the AbinitioRelax application as implemented in Rosetta 3.0 (ref. 13 ). This application resulted in 5,000 possible structures and only conformations in structural agreement with the initial estimate were used in the second stage of this procedure. We chose the structure that permitted the accommodation of the phosphate group in the S17 position without disturbing the structure of the peptide ( Supplementary Fig. S5a,b ). 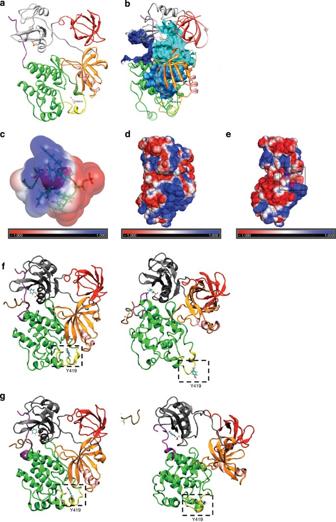Figure 4: Interaction between pS17 and Src results in conformational changes that expose Y419. (a) Inactive form of the protein obtained from the protein data bank (PDB code:2SRC). The ANP and all the water molecules were deleted from the PDB structure. (b) View of the three identified cavities where the peptide could be inserted. Charge distribution analysis of (c) designed model peptide, (d) Src and (e) the model peptide docked in the proposed cavity. The red and blue regions represent negative and positive charges, respectively. (f) After the phosphopeptide was exposed to Src for 36 ns, the kinase domain moved, completely exposing Y419. (g) When Src was exposed to an unphosphorylated peptide, no significant movement was observed and Y419 was not exposed. The SH3, SH2, N-lobe and alphaC domains are shown in red, grey, orange and pink, respectively. The C-lobe, A-loop, C-terminus and phosphopeptide are shown in green, yellow, purple and brown, respectively. Figure 4: Interaction between pS17 and Src results in conformational changes that expose Y419. ( a ) Inactive form of the protein obtained from the protein data bank (PDB code: 2SRC ). The ANP and all the water molecules were deleted from the PDB structure. ( b ) View of the three identified cavities where the peptide could be inserted. Charge distribution analysis of ( c ) designed model peptide, ( d ) Src and ( e ) the model peptide docked in the proposed cavity. The red and blue regions represent negative and positive charges, respectively. ( f ) After the phosphopeptide was exposed to Src for 36 ns, the kinase domain moved, completely exposing Y419. ( g ) When Src was exposed to an unphosphorylated peptide, no significant movement was observed and Y419 was not exposed. The SH3, SH2, N-lobe and alphaC domains are shown in red, grey, orange and pink, respectively. The C-lobe, A-loop, C-terminus and phosphopeptide are shown in green, yellow, purple and brown, respectively. Full size image To identify possible cavities in the structure of the protein where the peptide could interact, we subjected the inactive structure of c-Src to a Computed Atlas of Surface Topography of Proteins [14] analysis using the University of California at San Francisco Chimera interface. The obtained results suggested three possible cavities with an area and volume large enough to accommodate the designed peptide ( Fig. 4b and Supplementary Fig. S5c ). One of these cavities is the active site where ANP binds, which is not spatially accessible for the peptide until the protein is in its active conformation. To elucidate which of the cavities was the best candidate, the structure of Src was compared with the human tyrosine kinase c-Abl, (PDB code: 2fo0 ). Both of these structures were aligned using the Multiseq plug-in [15] in the Visual Molecular Dynamics package (VMD 1.8.4) [16] . c-Abl has a different auto-inactivation mechanism compared with c-Src. However, this mechanism involves interaction of the N-terminal Myristoyl group with the four major helices (H11, H16, H18 and H20) in the kinase domain. This structure includes residues 65–82 that are part of the N-terminal cap of c-Abl. Owing to the structural resemblance between Src and c-Abl (47% sequence homology) [17] , it is plausible that the conformation of the N-terminus in c-Abl is similar to the N-terminus in Src, and hence it is possible to conclude that the N-terminus of c-Src follows a similar trajectory as the N-terminus of c-Abl, a trajectory that is well known. On the basis of this analysis, Src has only one possible cavity where the peptide can be inserted. This cavity is located near the C-terminal, and between the SH2 and kinase domain ( Fig. 4b and Supplementary Fig. S5c ). This cavity is also the most accessible of the three cavities we identified. Furthermore, we used molecular dynamics to simulate a hydrated Src and performed solvation analyses [18] , [19] , [20] of the selected cavity to ensure that water displacement from the allosteric site is thermodynamically favourable. This approach identified eight high solvent density regions in the cavity that are thermodynamically unfavourable and displaced after the peptide binds. Water displacement from these regions to more thermodynamically favourable bulk biological fluid strongly suggests that the peptide can bind at this site ( Supplementary Fig. S5d ). As the peptide contains a high content of charged residues (63.6%), a charge distribution analysis was performed using the Adaptive Poisson–Boltzmann Solver within Pymol [21] , while the charges and radii used were obtained from the amber99SB force field [22] . Our results demonstrated that the chosen cavity had a highly negative charged surface in the interior that could accommodate the positive portion of the peptide while exhibiting a positively charged entrance that could accommodate the negative charge on the other part of the peptide ( Fig. 4c–e ). Hence, from an electrostatic point of view, this cavity provides the correct environment for protein–peptide interaction. Finally, we performed molecular dynamic simulations using the inactive structure of c-Src with the phosphorylated peptide docked to the cavity that we identified in our previous simulations. Our results demonstrate that the Src/phosphorylated peptide model undergoes significant structural changes in the kinase domain, that is, exposure of the Y419 residue without alteration of the C-terminus ( Fig. 4f , Supplementary Movie 1 ). Additionally, our simulation showed that the SH2 domain maintained its closed conformation. These two changes are characteristic of the activated form of Src. Supplementary Fig. S5e depicts a probability contour of the contacts between the phosphorylated peptide and the protein throughout the simulated timeframe. In contrast, a peptide containing a S17A mutation had a negligible difference in its polarity when compared to an unphosphorylated peptide and due to size of this system, we assumed this difference to be insignificant. Hence, we performed simulations of Src in the presence of a peptide lacking S17 phosphorylation. Furthermore, no significant alteration of the protein structure was observed when the simulation was run with this peptide ( Fig. 4g and Supplementary Movie 2 ). Moreover, during the simulated time, the unphosphorylated peptide leaves the cavity, suggesting that the interaction between the peptide and Src is not as strong as with the phosphorylated peptide. To confirm these results, we performed a kinase assay where Src was exposed to the same phosphorylated peptide used in our molecular dynamic simulations. Upon interaction with the phosphorylated peptide, Src Y419 phosphorylation was substantially elevated, resulting in enhanced enzymatic activity and increased Src-dependent FAK phosphorylation at Y861 ( Supplementary Fig. S5f–h ). Src mediates NA-induced cell migration and invasion To determine the functional effects of NA-induced Src S17 phosphorylation, we first examined its effects on cell migration. In WT Src-transfected SYF cells, NA increased S17 phosphorylation, while PDGF treatment did not ( Fig. 3d ). Furthermore, NA and PDGF treatment significantly increased migration of WT Src-transfected SYF cells ( P <0.01). In contrast, NA did not stimulate the migration of S17A Src-transfected SYF cells, while PDGF still promoted cell migration ( P <0.01; Fig. 3d ). In non-transfected SYF cells, NA failed to induce an increase in the migratory ability of these cells ( Supplementary Fig. S4i ). These data indicate that NA-induced Src activation requires direct phosphorylation of S17, which results in Src Y419 phosphorylation, a mechanism distinct from Src activation by classic growth factor/growth factor receptor interactions. To determine whether Src or PKA were responsible for mediating the stimulatory effects of catecholamines, we used three different Src siRNA sequences that silenced Src expression by >80%, AP23846 or KT5720 ( Supplementary Fig. S6a and data not shown). NA treatment significantly increased the invasive potential of SKOV3ip1 and HeyA8 cells ( P <0.01; Fig. 5a and Supplementary Fig. S6c,d ). Src siRNA or AP23846 completely abrogated the NA-induced increase in invasion in both cell lines ( Fig. 5a and Supplementary Fig. S6c ), while KT5720 blocked NA-induced invasion in SKOV3ip1 cells ( Supplementary Fig. S6d ). Furthermore, NA-induced migration of SKOV3ip1 or HeyA8 cells was abrogated with Src siRNA treatment or AP23846 ( Fig. 5b and Supplementary Fig. S6b ). Next, we used the poorly invasive A2780-ADRB2 cells because they express very low levels of Src when compared with a panel of ovarian cancer cells (data not shown). After transiently transfecting these cells with a vector carrying either WT Src or S17A Src, invasion assays were carried out. WT Src potentiated the effect of NA on the invasiveness of these cells, while the introduction of S17A Src failed to have a similar effect when compared with non-transfected A2780-ADRB2 cells ( Supplementary Fig. S6e ). Additionally, we transfected ID8 VEGF murine ovarian carcinoma cells with human WT Src or S17A Src and then silenced endogenous Src by treating them with siRNA targeted against murine Src. Cells were then exposed to NA and subjected to migration and invasion assays. NA treatment resulted in increased cancer cell migration and invasion in WT Src-ID8 VEGF cells, but not in the S17A Src-ID8 VEGF cells ( Supplementary Fig. S6f,g ). 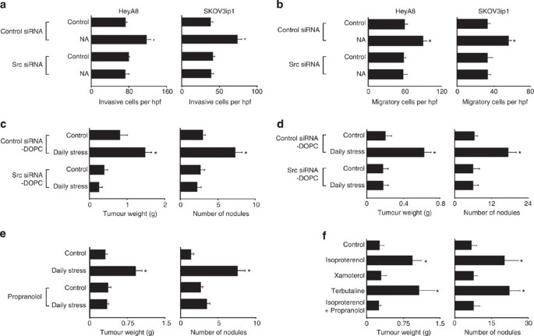Figure 5: Adrenergic-mediated Src activation leads to increased tumour invasion and growth. NA 10 μM induces HeyA8 and SKOV3ip1 (a) cell invasion and (b) migration. (c) Mice were inoculated with either HeyA8 (2.5 × 105) or (d) SKOV3ip1 (1.0 × 106) cells and subjected to daily restraint and treated twice a week with either control siRNA-DOPC or Src siRNA-DOPC. Treatment with Src siRNA-DOPC blocked the daily restraint-mediated induction in tumour weight and number of nodules compared with control siRNA-DOPC. (e) Mice bearing SKOV3ip1 tumours undergoing daily restraint were treated daily with propranolol (2 mg kg−1). Propranolol counteracts the effects of daily restraint on tumour growth. (f) Mice bearing SKOV3ip1 tumours were treated daily with either: 10 mg kg−1isoproterenol, 5 mg kg−1terbutaline, 1 mg kg−1xamoterol or isoproterenol plus 2 mg kg−1of propranolol. Isoproterenol and terbutaline induced tumour growth, but not xamoterol. Mice treated with isoproterenol plus propranolol have tumour burden similar to control mice. Figure 5: Adrenergic-mediated Src activation leads to increased tumour invasion and growth. NA 10 μM induces HeyA8 and SKOV3ip1 ( a ) cell invasion and ( b ) migration. ( c ) Mice were inoculated with either HeyA8 (2.5 × 10 5 ) or ( d ) SKOV3ip1 (1.0 × 10 6 ) cells and subjected to daily restraint and treated twice a week with either control siRNA-DOPC or Src siRNA-DOPC. Treatment with Src siRNA-DOPC blocked the daily restraint-mediated induction in tumour weight and number of nodules compared with control siRNA-DOPC. ( e ) Mice bearing SKOV3ip1 tumours undergoing daily restraint were treated daily with propranolol (2 mg kg −1 ). Propranolol counteracts the effects of daily restraint on tumour growth. ( f ) Mice bearing SKOV3ip1 tumours were treated daily with either: 10 mg kg −1 isoproterenol, 5 mg kg −1 terbutaline, 1 mg kg −1 xamoterol or isoproterenol plus 2 mg kg −1 of propranolol. Isoproterenol and terbutaline induced tumour growth, but not xamoterol. Mice treated with isoproterenol plus propranolol have tumour burden similar to control mice. Full size image We next asked if an increase in Src activity, upon adrenergic stimulation, could result in the induction of genes known to be mediators of cell motility and invasion. To address this question, we performed a cDNA microarray analysis of NA-treated SKOV3ip1 cells and identified genes relevant for tumour cell invasion. Our analysis revealed a significant increase in several such genes following NA treatment, and this increase was blocked by Src silencing ( Supplementary Fig. S6h ). Restraint stress-induced tumour growth is mediated by Src To test the biological significance of adrenergic-mediated Src activation, we utilized an in vivo restraint stress model [2] . In this model, tumours from animals exposed to daily restraint had substantially increased levels of pSrc Y419 ( Supplementary Fig. S7b ) compared with controls. Src siRNA was incorporated into 1,2-dioleoyl-sn-glycero-3-phosphatidylcholine (DOPC) nanoliposomes for in vivo delivery. After confirming >80% reduction in Src levels in vivo ( Supplementary Fig. S7a ), we treated control or restrained mice ( n =10 per group) bearing SKOV3ip1 or HeyA8 tumours with control siRNA-DOPC or Src siRNA-DOPC. As expected, daily restraint significantly increased tumour growth ( Fig. 5c ). This increase was completely blocked by Src siRNA-DOPC ( Fig. 5c ). Furthermore, the number of tumour nodules was also reduced by Src siRNA-DOPC in both the HeyA8 and SKOV3ip1 models ( Fig. 5c ). These results were confirmed by additional experiments that utilized two different Src-specific siRNA sequences and the Src small molecule inhibitor, AP23846 ( Supplementary Fig. S7c,d ). Next, we analysed tumour tissues from daily restraint versus control mice that were treated with control siRNA or Src-specific siRNA with the proliferation markers phospho-histone h3 and proliferating cell nuclear antigen and the apoptotic marker cleaved caspase 3. Restraint stress resulted in increased cell proliferation that was abrogated by Src siRNA treatment ( Supplementary Fig. S7e,f ). There were no significant changes in apoptosis between any groups (data not shown). As our data indicate that increased adrenergic signalling results in increased invasion in vitro , we analysed H&E sections obtained from tumour bearing mice undergoing restraint stress. These results show that restraint stress leads to tumour infiltration into underlying tissue and Src siRNA-DOPC abrogates this effect ( Supplementary Fig. S7g ). Moreover, we found that tumours from mice undergoing restraint stress had elevated β-catenin levels, while Src siRNA-DOPC blocks this increase ( Supplementary Fig. S7h ). To determine the contribution of ADRB in the daily restraint model, we treated control or restrained mice ( n =10 per group) bearing HeyA8 tumours with propranolol. As expected, propranolol abrogated the daily restraint-induced increase in tumour growth ( Fig. 5e ). Tumours from animals treated with propranolol and exposed to daily restraint stress had substantially decreased levels of pSrc Y419 compared with mice exposed to daily restraint stress ( Supplementary Fig. S7i ). To further delineate the role of ADRB on tumour growth, we treated HeyA8 tumour bearing mice ( n =10 mice) with either isoproterenol, xamoterol, terbutaline or isoproterenol plus propranolol. As expected, isoproterenol significantly increased tumour growth, and a similar increase in tumour burden was noted with terbutaline ( Fig. 5f ). However, treatment with xamoterol or propranolol in combination with isoproterenol did not result in increased tumour growth compared with the control group ( Fig. 5f ). Tumours from animals exposed to isoproterenol or terbutaline had substantially increased levels of pSrc Y419 and pSrc S17 , while xamoterol or propranolol in combination with isoproterenol did not induce phosphorylation at these sites ( Supplementary Fig. S7j ). Additionally, bioluminescence imaging analysis revealed that daily restraint stress resulted in significantly increased tumour growth and metastasis, which was abrogated by the use of propranolol ( Supplementary Fig. S7k ). Next, to determine the effects of daily restraint stress on the patterns of metastasis, we utilized a fully orthotopic mouse. SKOV3ip1 ovarian cancer cells were injected directly into the right ovary of nude mice followed by exposure to daily restraint stress, with or without Src siRNA-DOPC treatment. Daily restraint stress resulted in significantly higher tumour nodule counts and distant metastatic spread compared with control siRNA-DOPC ( Supplementary Fig. S7l ). Src siRNA-DOPC completely abrogated the effects of stress on tumour metastasis ( Supplementary Fig. S7l ). To further delineate the role of ADRB2 in vivo , we inoculated mice ( n =7 per group) with A2780-OG2 (empty vector), A2780-ADRB2 or A2780 cells into the subcutaneous space and treated groups with isoproterenol or PBS. Isoproterenol significantly increased tumour growth in the A2780-ADRB2 group compared with the A2780-OG2 group, whereas the A2780 group did not respond to isoproterenol treatment ( Supplementary Fig. S7m ). To examine the role of increased peripheral nervous system activity on tumour growth, we performed an experiment where mice undergoing daily restraint stress were inoculated with SKOV3ip1 cells and treated with the peripheral ganglionic blocker hexamethonium bromide (daily dose of 1 mg kg −1 ). This treatment completely blocked the daily restraint-induced tumour growth (data not shown). Next, we used ID8 VEGF murine ovarian cancer cells transfected with human WT Src or S17A mutated Src. These cells were then injected subcutaneously into the right flank of C57 mice, treated with murine Src siRNA-DOPC (to silence endogenous Src; Supplementary Fig. S7n ) and isoproterenol. Isoproterenol treatment resulted in significantly increased tumour growth in mice inoculated with WT Src-cells, but not with S17A Src-cells ( Supplementary Fig. S7n ). pSrc Y419 expression in human ovarian carcinoma To determine whether adrenergic activity might relate to Src activation in human cancers, we examined 91 invasive epithelial ovarian cancers. Consistent with prior reports [23] , [24] , increased Src expression was noted in 88% of the tumour samples, while elevated pSrc Y419 expression was noted in 42% ( Fig. 6a ). We found that elevated levels of pSrc Y419 were associated with poor mean patient survival by univariate analysis (1.67 years versus not yet reached; P <0.001; Fig. 6b ). As depression, as measured by high scores on the Centre for Epidemiological Studies Depression scale (CES-D) [25] , [26] , has been linked to increased tumour catecholamine levels [27] , [28] , we examined potential relationships between CESD scores and Src activity. Patients with high CES-D scores (≥16) had significantly higher levels of tumoural pSrc Y419 ( P =0.008) compared with those with low scores ( Fig. 6c ). In addition, NA levels above the median were significantly associated with increased pSrc Y419 expression ( P <0.001), but not with increases in total Src ( Fig. 6c ). In a subset of these tumour samples, pSrc Y419 and pSrc S17 levels were evaluated by ELISA and western blot analyses, respectively. There was a significant association between elevated pSrc Y419 and pSrc S17 in these samples ( Supplementary Fig. S8a ). Moreover, we found a strong positive correlation between tumoural NA and pSrc Y419 and pSrc S17 levels ( Supplementary Fig. S8b,c ). 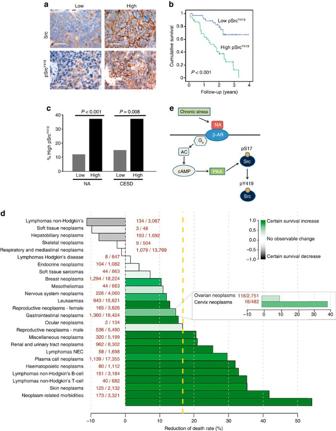Figure 6: High pSrcY419levels are associated with decreased survival and depressive symptoms. (a) Representative images of human ovarian tumours with low or high expression of Src and pSrcY419. Images were taken at original magnification X200 (scale bar=50 μm). (b) Kaplan-Meier curves of disease-specific mortality for patients with epithelial ovarian carcinoma (n=91) based on pSrcY419expression. The log-rank test (two-sided) was used to compare differences between groups. (c) Percentage of ovarian cancers with high pSrcY419expression based on tumoural NA levels (greater than the median value of 0.84 pg mg−1versus less than 0.84 pg mg−1) and CESD scores ≥16. (d) Effect of beta blocker usage on cancer-related mortality, as estimated based on data from the FDA Adverse Event Reporting System. Bars, mortality decrease (green) or increase (black) by cancer type; saturation representing statistical confidence. Dashed yellow line, general mortality reduction over all cancer-related cases (17%). Numbers, cases having received a beta-blocker/total number of cases with given cancer type. (e) In response to chronic stress, catecholamines are released from the sympathetic nervous system. Stress-related hormones bind and activate ADRB receptors on tumour cells, initiating a cascade of events that result in Src activation. Figure 6: High pSrc Y419 levels are associated with decreased survival and depressive symptoms. ( a ) Representative images of human ovarian tumours with low or high expression of Src and pSrc Y419 . Images were taken at original magnification X200 (scale bar=50 μm). ( b ) Kaplan-Meier curves of disease-specific mortality for patients with epithelial ovarian carcinoma ( n =91) based on pSrc Y419 expression. The log-rank test (two-sided) was used to compare differences between groups. ( c ) Percentage of ovarian cancers with high pSrc Y419 expression based on tumoural NA levels (greater than the median value of 0.84 pg mg −1 versus less than 0.84 pg mg −1 ) and CESD scores ≥16. ( d ) Effect of beta blocker usage on cancer-related mortality, as estimated based on data from the FDA Adverse Event Reporting System. Bars, mortality decrease (green) or increase (black) by cancer type; saturation representing statistical confidence. Dashed yellow line, general mortality reduction over all cancer-related cases (17%). Numbers, cases having received a beta-blocker/total number of cases with given cancer type. ( e ) In response to chronic stress, catecholamines are released from the sympathetic nervous system. Stress-related hormones bind and activate ADRB receptors on tumour cells, initiating a cascade of events that result in Src activation. Full size image Beta blockers may reduce cancer-related mortality To examine the potential clinical impact of our findings, we asked whether chemical perturbation of beta-adrenergic function in cancer patients might result in lower patient mortality. To test this hypothesis, we employed adverse events data from the FDA’s Adverse Event Reporting System (AERS; http://www.fda.gov/Drugs/GuidanceComplianceRegulatoryInformation/Surveillance ) to examine whether usage of beta blockers by patients affected cancer-related mortality. Our analysis revealed that mortality (that is, ‘Death’ reported either as a patient’s outcome or as a patient’ reaction), was reduced by an average of 17% across all major cancer types if patients were treated with beta blockers ( Fig. 6d ). Moreover, a 14.64% decrease in mortality was observed among patients with ovarian and cervical cancer. These data suggest that beta blocker use among cancer patients can significantly reduce cancer-related mortality. Here, we describe a unique mechanism by which increased adrenergic signalling results in Src activation, which induces downstream proteins important for cell survival, motility and invasion [29] , [30] , [31] . Increased serine phosphorylation at Src amino terminus following cAMP treatment was demonstrated 30 years ago [32] , and a consensus PKA site at Src S17 was subsequently identified [33] . However, no physiological role for phosphorylation at Src S17 had been established; pSrc S17 can mediate Rap1 activation and inhibit ERK by cAMP-dependent pathways [34] , [35] . Src has been implicated in NA-stimulated VEGF production by adipocytes [36] , [37] , and in NA-stimulated IL-6 production by cancer cells [7] . Although different mechanisms have been suggested to account for ADRB-mediated Src activation (for example, β-arrestin and EGFR-dependent Src phosphorylation [38] ), the precise mechanisms mediating ADRB/cAMP/PKA-induced Src activation or the resultant biological effects were not well understood. Our results have identified a new functional role for Src S17 as a key molecular switch that links a serine kinase to downstream tyrosine kinase signalling and disease progression ( Fig. 6e ). Specifically, our results indicate that the neuroendocrine stress response can directly affect tumour growth and malignant progression through receptors expressed on tumour cells that lead to a critical phosphorylation event, resulting in Src activation. NA is the most abundant stress hormone in the ovary [39] , [40] and its levels are much higher in the ovary than in the plasma [41] , [42] . To the extent that biobehavioral states can modulate catecholamine levels in the tumour microenvironment, these findings offer new opportunities for designing interventions to protect individuals from the harmful effects of chronic adrenergic stimulation [43] . A number of studies have recently emerged supporting the rationale for designing clinical studies to target neuroendocrine function, which could represent a new avenue for treating individuals with cancer [44] . On the basis of our work, beta-antagonists can abrogate many of the deleterious effects of increased adrenergic signalling. For example, among prostate cancer patients taking anti-hypertensive medication, only beta blockers were associated with a reduction of cancer risk [44] , while others have shown a reduction in overall cancer risk [45] . Moreover, our findings support the use of Src family kinase inhibitors as tools to block the deleterious effects of increased sympathetic activity [46] , [47] . Collectively, our data represent a new understanding of Src regulation in response to adrenergic signalling in cancer cells and provide a biologically plausible and potent way of inhibiting tumour progression among cancer patients. Proteomic analysis Two-dimensional gel electrophoresis was conducted as first described by O’Farrell [48] . All biological samples were run in duplicate (technical). After electrophoresis, the gels were fixed and either directly stained with SYPRO-Rube (Bio-Rad, Hercules, CA) or sequentially stained with ProQ-Diamond (detects phosphate groups attached to tyrosine, serine or threonine residues) and SYPRO-Ruby (detects total protein). Gels were then scanned at a 100-mm resolution using the Perkin-Elmer ProEXPRESS 2D Proteomic Imaging System (Boston, MA). After quantifying the relative spot intensities among samples and normalizing the phosphorylation levels to the total amount of protein, gel spots were excised and prepared for MALDI-TOF-MS analysis using DigiLab’s (Holliston, MO) ProPic and ProPrep robotic instruments following the manufacturer’s protocol. MALDI-TOF/TOF was performed using the Applied Biosystems 4800 MALDI TOF/TOF analyser for peptide mass fingerprinting and sequencing (See Supplementary Procedures for a more detailed description). Protein identification was performed using a Bayesian algorithm, where high probability matches are indicated by an expectation score, which is an estimate of the number of matches that would be expected in that database if the matches were completely random [49] . See Supplementary Procedures for expanded methodology. Signalling network analysis We sought to analyse whether a key mediator kinase might exist that is capable of directly or indirectly explaining the majority of the observed differences in phosphorylation and protein abundance. We restricted the length of signalling chains to include at most two phosphorylation events (equivalently, allowing for at most one intermediate kinase, because otherwise, the set of potential candidates would suffer from ‘combinatorial explosion’). We constructed this two-layer phosphorylation network upstream of the identified proteins using information from Phospho.ELM and networKIN [50] , [51] . In the resultant network, 45 of the dysregulated proteins could be linked to at least one of 243 kinases. Scoring and sorting these candidates by the number of downstream dysregulated proteins suggested Src as a tentative key mediator for the experimentally observed differences (37/45 proteins, Fig. 1 and Supplementary Fig. S2a ). We note that this neither disproves an important role for other kinases nor proves that Src is the most important kinase in this context; however, it does illustrate some potential for Src being of central importance in the cellular response to NA. Western blot analysis Cell lysates were prepared by washing cells with phosphate-buffered saline and incubating them for 10 min at 4 °C in modified radioimmunoprecipitation assay lysis buffer. Cells were scraped from plates and centrifuged for 20 min at 4 °C, and the supernatant was collected. Protein concentrations were determined using a BCA reagent kit (Pierce), and 40 μg of whole-cell lysates were separated by 10% SDS–PAGE. Samples were transferred to a nitrocellulose membrane by wet electrophoresis (Bio-Rad), blocked with 5% nonfat milk for 1 h at room temperature, and incubated with Src, pSrc Y416 , pSrc S17 or pSrc Y530 overnight at 4 °C. Primary antibody was detected with anti-rabbit IgG (Amersham Biosciences, Piscataway, NJ) and developed with an enhanced chemiluminescence detection kit (Pierce, Rockford, IL). siRNA preparation and treatment We used siRNA to downregulate Src in vitro and in vivo . Src-specific siRNA was purchased from Ambion (Austin, TX) with the following target sequence: 5′-GGCTGAGGAGTGGTATTTT-3′. Additional validated Src sequences were purchased from Sigma-Genosys (The Woodlands, TX). Control siRNA used was obtained from Qiagen (Valencia, CA) with the following target sequence: 5′-AATTCTCCGAACGTGTCACGT-3′. For in vitro studies, cells were transfected with siRNA that was incorporated into Lipofectamine 2000 transfection reagent (Invitrogen, Carlsbad, CA) following the manufacturer’s protocol. After 72 h, the experiments were carried out. For in vivo studies, siRNA was incorporated into the neutral liposome DOPC as previously described [52] , [53] . For each treatment, 3.5 μg of siRNA was reconstituted in 200 μl of phosphate-buffered saline and administered by intravenous injection. The dosing schedule is described in the in vivo tumour model below. Migration and invasion assay The membrane invasion culture system chamber was used to measure the in vitro invasive and migratory potential of all cell lines used in this study. When required, siRNA was added to cells 24 h before cell harvest, and NA was added at the start of the experiment. The membrane invasion culture system assay was performed as previously described. Briefly, single cell tumour suspensions were seeded into the upper wells at a concentration of 1 × 10 5 cells per well for the invasion assays and 7.5 × 10 4 cells per well for the migration assays. For the invasion and migration assays, a human basement membrane and gelatin-coated membrane were used, respectively. Cells were allowed to invade for 24 h or migrate for 6 h for the invasion and migration assays, respectively. The cells were then collected, fixed, stained and counted by light microscopy. Chronic stress model We obtained 8- to 12-week-old female athymic nude mice from the National Cancer Institute. All experiments were approved by the Institutional Animal Care and Use Committee at MD Anderson Cancer Center. To experimentally induce stress in the mice, we used a restraint-stress procedure that utilizes a physical restraint system that we developed. Tumour cells were injected intraperitoneally or subcutaneously into mice in all groups 7 days after the stress procedure began. A total of 10 mice per group were used. Starting 4 days after tumour cell injection, mice were treated with siRNA (control or Src-specific, 3.5 μg in DOPC every 3 days, intraperitoneally) for the duration of the experiments. We necropsied the animals 21 days after tumour cell injection. At this time, the entire peritoneal cavity was examined for identifiable disease, and mouse weight, tumour weight and the distribution of tumour was recorded by gynaecological oncologists. Centre for epidemiological studies depression scale Patients completed psychosocial questionnaires between their initial preoperative appointment and surgery. The CES-D scale is a 20-item measure that assesses depressive symptomatology over the last week [25] . Scores of 16 or higher have been associated with clinical depression. Statistical analysis We compared continuous variables using either Student’s t -test or analysis of variance and compared the categorical variables using the χ 2 -test. We used a nonparametric test (Mann–Whitney test), when appropriate, to compare differences. We considered P <0.05 to be significant. Additional methods Details of reagents, cell culture conditions, mass spectrometry, protein identification analysis, microarray analysis, plasmids, kinase assay, immunochemistry, immunoprecipitation and methods used to determine NA concentration, molecular dynamic simulations and the bioinformatics analysis of the FDA adverse event reports can be found in the Supplementary Methods . How to cite this article: Armaiz-Pena, G. N. et al. Src activation by β-adrenoreceptors is a key switch for tumor metastasis. Nat. Commun. 4:1403 doi: 10.1038/ncomms2413 (2013).